Quantum dynamics of CO–H2in full dimensionality Accurate rate coefficients for molecular vibrational transitions due to collisions with H 2 , critical for interpreting infrared astronomical observations, are lacking for most molecules. Quantum calculations are the primary source of such data, but reliable values that consider all internal degrees of freedom of the collision complex have only been reported for H 2 -H 2 due to the difficulty of the computations. Here we present essentially exact, full-dimensional dynamics computations for rovibrational quenching of CO due to H 2 impact. Using a high-level six-dimensional potential surface, time-independent scattering calculations, within a full angular momentum coupling formulation, were performed for the de-excitation of vibrationally excited CO. Agreement with experimentally determined results confirms the accuracy of the potential and scattering computations, representing the largest of such calculations performed to date. This investigation advances computational quantum dynamical studies representing initial steps towards obtaining CO–H 2 rovibrational quenching data needed for astrophysical modelling. Quantum mechanical studies of inelastic processes in molecular collisions began with the development of the nearly exact, close-coupling (CC) method for rotational transitions in atom–diatom collisions by Arthurs and Dalgarno [1] and Takayanagi [2] in the 1960s. Over the past five decades tremendous advances in computational processing power and numerical algorithms have allowed high-level computations of inelastic processes [3] , [4] , as well as reactive collisional dynamics of large molecular systems, the latter using primarily time-dependent approaches [5] , [6] , [7] . Until recently, however, the largest full-dimensional inelastic studies for a system of two colliding molecules have been limited to H 2 -H 2 collisions in six-dimensions (6D), which were performed with both time-independent [8] and time-dependent [9] , [10] approaches for solving the Schrödinger equation. However, to make these computations possible, the authors resorted to various angular-momentum decoupling approximations with uncertain reliability. It was only recently [11] , [12] , [13] that these decoupling approximations were relaxed and essentially exact full-dimensional CC computations for the H 2 -H 2 system became feasible. Despite the large internal energy spacing of H 2 , which allows the basis sets to be relatively compact, these calculations are computationally demanding. Replacing one H 2 molecule with a molecule that has smaller internal energy spacing, such as carbon monoxide, would further increase the computational demands. Whether the CC method could in practice be used to describe such a diatom–diatom system in full dimensionality remains an open question. First detected in the interstellar medium in 1970 (ref. 14 ), carbon monoxide is the second most abundant molecule, after H 2 , in most astrophysical environments. CO has been the focus of countless theoretical astrophysical studies and observations, being detected in objects as distant as high redshift quasars [15] to cometary comae in our solar system [16] to the atmospheres of extrasolar giant planets [17] . Most studies have focused on pure rotational transitions observed in the far infrared to the radio or electronic absorption in the near ultraviolet. Over the past decade, however, near infrared emission of CO due to the fundamental vibrational band near 4.7 μm has been detected in a variety of sources including star-forming regions in Orion with the Infrared Space Observatory [18] and protoplanetary disks (PPDs) of young stellar objects [19] , [20] , [21] with the Gemini Observatory and the Very Large Telescope. In addition, pure rotational transitions, but in the first two vibrationally excited states ( v 1 =1 and 2), were detected by the Submillimeter Array in the circumstellar shell of the much-studied evolved star IRC+10216 (ref. 22 ). In particular, high-resolution observations of the CO fundamental band probe the physical conditions in the inner disk region, ~10–20 astronomical units (AU), the site of planet formation. Detailed modelling of such environments requires state-to-state inelastic rovibrational excitation rate coefficients for CO due to H 2 collisions, but current simulations are limited to approximate scaling methods due to the dearth of explicit data [18] , [23] . In this Article, we address the two issues outlined above by advancing the state-of-the-art for inelastic quantum dynamics with a full-dimensional investigation using an accurate potential energy surface (PES) relevant to this scattering process, with a particular emphasis on the important region of the van der Waals complex. This was made possible through the accurate computation and precise fitting of a 6D CO–H 2 PES in the relevant region of the formaldehyde tetra-atomic system and the further development of the inelastic diatom–diatom time-independent scattering code, TwoBC [24] , which performs full angular momentum coupling, the CC formalism [1] , including vibrational degrees of freedom. We first briefly describe the new CO–H 2 PES and its testing through comparison of rotational excitation calculations using the 6D PES and 4D PESs (neglecting vibrational motion) and available experimental results. The full-dimensional (6D), essentially exact, computations for rovibrational quenching of CO( v 1 = 1) due to H 2 collisions are presented resolving a two-orders-magnitude discrepancy between earlier 4D calculations, which adopted various approximations [25] , [26] , [27] , [28] . Finally, the current results are shown to be consistent with the rovibrational quenching measurements for the CO–H 2 system, performed at the Oxford Physical Chemistry Laboratory from 1976–1993, which no prior calculation has yet been able to adequately explain [29] , [30] , [31] . The CO–H 2 PES The CO–H 2 interaction has been of considerable interest to the chemical physics community for many decades with one of the first 4D surfaces for the electronic ground state constructed by Schinke et al . [32] , which was later extended by Baĉić et al . [25] The group of Jankowski and Szalewicz [33] performed accurate 5D and 6D electronic energy calculations, but averaged over monomer vibrational modes, and performed several fits to obtain a series of 4D rigid-rotor surfaces, referred to as the V98 (ref. 33 ), V04 (ref. 34 ) and V12 (ref. 35 ) PESs. A 6D PES for formaldehyde was constructed earlier by Zhang et al . [36] , but it was developed for reactive scattering applications and, consequently, limited attention was given to the long-range CO–H 2 van der Waals configuration. Therefore, as a prerequisite to 6D inelastic dynamics studies, we carried out an unprecedented potential energy calculation including over 459 756 energy points (see Methods for details). The potential energy data were then fit using the invariant polynomial method with Morse-type variables in terms of bond-distances [37] , [38] . The resulting 6D PES, referred to as V6D, is shown in Fig. 1 for one sample configuration. Some features of V6D are also illustrated in Supplementary Figs 2–4 . 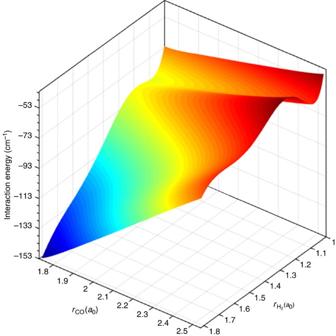Figure 1: The CO–H2interaction potential energy surface V6D. The potential surface is constructed in the 6D diatom–diatom Jacobi coordinates (R,r1,r2,θ1,θ2,φ),r1andr2are bond lengths,Rthe internuclear distance between CO and H2centre of masses,θ1andθ2the angles betweenRandr1andr2, andφthe dihedral or twist angle. SeeSupplementary Figure 1. Here the dependence of the potential surface on bond lengthsrCO=r1andrH2=r2is shown withR=8 a0,θ1=180°,θ2=0 andφ= 0. Note that the CO(r1) and H2(r2) diatom potentials have been subtracted. Figure 1: The CO–H 2 interaction potential energy surface V6D. The potential surface is constructed in the 6D diatom–diatom Jacobi coordinates ( R , r 1 , r 2 , θ 1 , θ 2 , φ ), r 1 and r 2 are bond lengths, R the internuclear distance between CO and H 2 centre of masses, θ 1 and θ 2 the angles between R and r 1 and r 2 , and φ the dihedral or twist angle. See Supplementary Figure 1 . Here the dependence of the potential surface on bond lengths r CO = r 1 and r H2 = r 2 is shown with R =8 a 0 , θ 1 =180°, θ 2 =0 and φ = 0. Note that the CO( r 1 ) and H 2 ( r 2 ) diatom potentials have been subtracted. Full size image Cross-sections and rate coefficients Time-independent quantum scattering calculations were performed using the CC formulation of Arthurs and Dalgarno [1] as implemented for diatom–diatom collisions in the 4D rigid-rotor approximation in MOLSCAT [39] and extended to full-dimensional dynamics as described by Quéméner, Balakrishnan, and coworkers [12] , [13] in TwoBC. In the first set of scattering calculations, the new 6D PES was tested for pure rotational excitation from CO( v 1 =0, j 1 =0,1), where v 1 and j 1 are the vibrational and rotational quantum numbers, respectively. The crossed molecular beam experiment of Antonova et al . [40] , who obtained relative state-to-state rotational inelastic cross-sections, is used as a benchmark. The experimental cross-sections were determined at three centre of mass kinetic energies (795, 860 and 991 cm −1 ), but with an initial state distribution of CO estimated to be 75±5% for j 1 =0 and 25±5% for j 1 =1. Antonova et al . [40] normalized the relative cross-sections to rigid-rotor calculations done with MOLSCAT using the V04 PES of Jankowski and Szalewicz [33] . Comparison of the experiment with new 4D rigid-rotor calculations on V12 and full-dimensional calculations on V6D are shown in Fig. 2 . We find no difference in the excitation cross-sections when using V04 or V12, while the root mean square (RMS) cross-section errors between the normalized experiment and the V12 and V6D calculations range from 0.56–0.89 × 10 −16 cm 2 to 0.55–0.95 × 10 −16 cm 2 , respectively (See Supplementary Table 1 and Supplementary Note 1 ). Clearly, a 4D rigid-rotor treatment of the dynamics is sufficient for describing rotational excitation at these relatively high energies. 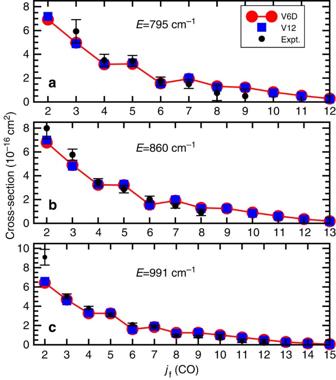Figure 2: State-to-state cross-sections for rotational excitation of CO(v1=0,j1=0,1) by collisions with H2. Theoretical results of full-dimensional calculations on V6D and 4D rigid-rotor calculations on V12 are compared with normalized experimental results40for collision energies of (a) 795 cm−1, (b) 860 cm−1and (c) 991 cm−1. The calculations were performed for H2(v2=0,j2=0), but the experimental H2rotational distribution was undetermined. The error bars correspond to twice the estimated s.d. in the weighted means of the measurements40. Figure 2: State-to-state cross-sections for rotational excitation of CO( v 1 =0, j 1 =0,1) by collisions with H 2 . Theoretical results of full-dimensional calculations on V6D and 4D rigid-rotor calculations on V12 are compared with normalized experimental results [40] for collision energies of ( a ) 795 cm −1 , ( b ) 860 cm −1 and ( c ) 991 cm −1 . The calculations were performed for H 2 ( v 2 =0, j 2 =0), but the experimental H 2 rotational distribution was undetermined. The error bars correspond to twice the estimated s.d. in the weighted means of the measurements [40] . Full size image The importance of full dimensionality for rotational excitation becomes more evident as the collision energy is reduced (see also Supplementary Figs 5 and 6 ). Low-energy excitation cross-sections for the process or (0000)→(0100), using the notation defined in Methods, were measured by Chefdeville et al . [41] in a crossed-beam experiment. They obtained the excitation cross-section for centre of mass kinetic energies from 3.3 to 22.5 cm −1 . Although their energy resolution was limited, three broad features were detected near 6, 13 and 16 cm −1 attributed to orbiting resonances. Computed cross-sections for process (1) using the 4D V12 PES and the full-dimensional V6D PES are presented in Fig. 3a . While both computations reveal numerous resonances, the resonances are generally shifted by 2-3 cm −1 between calculations. The energy and magnitude of the resonances are very sensitive to the details of the PESs, but differences may also be due to the relaxation of the rigid-rotor approximation with the use of V6D in TwoBC. In Fig. 3b , the two calculations are convolved over the experimental energy resolution and compared with the measured relative cross-sections. Except for the peak near 8 cm −1 , the current 6D calculation appears to reproduce the main features of the experiment. RMS errors are found to be 0.355 and 0.228 × 10 −16 cm 2 for the V12 and V6D PESs, respectively. Further details on the rotational excitation calculations can be found in Supplementary Note 1 . 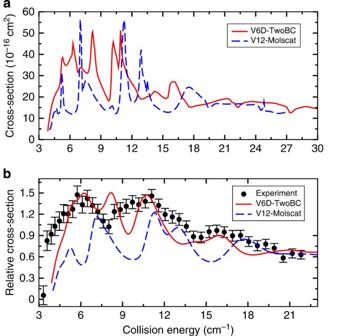Figure 3: Low-energy excitation cross-sections. j1=0 → 1 cross-sections for CO(v1=0) due to collisions with H2(v2=0,j2=0) are shown as a function of collision energy. (a) Computed cross-sections using the 4D V12 and 6D V6D PESs. (b) Computed cross-sections convolved over the experimental beam energy spread (lines) compared with the relative experiment of Chefdevilleet al.41(circles with error bars). The error bars on the experimental cross-sections of Chefdevilleet al. represent the statistical uncertainty at a 95% confidence interval. Figure 3: Low-energy excitation cross-sections. j 1 =0 → 1 cross-sections for CO( v 1 =0) due to collisions with H 2 ( v 2 =0, j 2 =0) are shown as a function of collision energy. ( a ) Computed cross-sections using the 4D V12 and 6D V6D PESs. ( b ) Computed cross-sections convolved over the experimental beam energy spread (lines) compared with the relative experiment of Chefdeville et al . [41] (circles with error bars). The error bars on the experimental cross-sections of Chefdeville et al . represent the statistical uncertainty at a 95% confidence interval. Full size image Now that the improved performance of the V6D potential for pure rotational excitation is apparent, we turn to rovibrational transitions. As far as we are aware, previous experimental [29] , [30] , [31] , [42] , [43] and theoretical [25] , [26] , [27] , [28] studies are limited to the total quenching of CO( v 1 =1). In the scattering calculations of both Baĉić et al . [25] , [26] and Reid et al . [27] , the 4D potential of Baĉić et al . [25] was adopted, in which two coordinates were fixed ( r 2 =1.4 a 0 , φ = 0), and various combinations of angular-momentum decoupling approximations for the dynamics were utilized (for example, the infinite order sudden, IOS, and coupled-states, CS, approximations; see Supplementary Note 2 ). More recently, Flower [28] performed CC calculations on a parameterization of the 4D PES of Kobaysashi et al . [44] These four sets of 4D calculations for quenching due to para-H 2 ( j 2 =0) are compared in Fig. 4 with the current 6D/CC calculations on the V6D surface for the case of . Corresponding state-to-state and total cross-sections for collisions with ortho-H 2 are given in Supplementary Figs 7–9 with further details in Supplementary Note 2 . 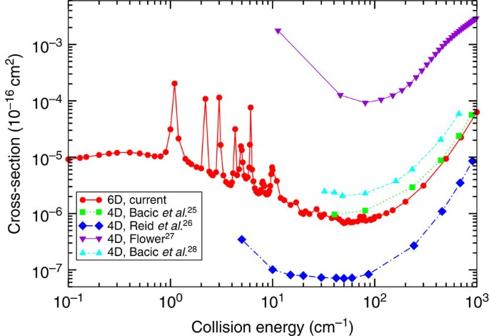Figure 4: Total theoretical cross-sections for the vibrational de-excitation of CO(v1=1) by para-H2. Current 6D/CC results are compared with previous 4D calculations. The 4D results of Baĉićet al.26and Reidet al.27do not distinguish CO rotational states, while the 4D results of Baĉićet al.25, 4D results of Flower28, and the current 6D/CC results are for initialj1=0 summed over all final CO(). In every case, the H2rovibrational state remains unchanged,. Figure 4: Total theoretical cross-sections for the vibrational de-excitation of CO( v 1 =1) by para-H 2 . Current 6D/CC results are compared with previous 4D calculations. The 4D results of Baĉić et al . [26] and Reid et al . [27] do not distinguish CO rotational states, while the 4D results of Baĉić et al . [25] , 4D results of Flower [28] , and the current 6D/CC results are for initial j 1 =0 summed over all final CO( ). In every case, the H 2 rovibrational state remains unchanged, . Full size image A cursory glance at Fig. 4 reveals a more than two-orders-of-magnitude discrepancy among the various calculations. The large dispersion for the previous calculations is due to a combination of reduced dimensionality and decoupled angular momentum, which makes it difficult to assess the reliability of each approximation. The current results, however, remove these uncertainties by utilizing (i) a full-dimensional (6D) PES, (ii) full-dimensional (6D) dynamics and (iii) full angular momentum coupling. The sharp peaks in the cross-sections over the 1–10 cm −1 range in the 6D/CC results are due to resonances [45] , [46] supported by the CO–H 2 van der Waals potential well. These resonances, in the rovibrational quenching of CO by H 2 , are reported here for the first time and their prediction is made possible through our high-level treatment of the dynamics. Computations for transitions involving other initially excited j 2 states and inelastic H 2 ( ) transitions are presented and compared in Supplementary Figs 10 and 11 and Supplementary Note 2 . Using the current 6D/CC cross-sections and the 4D/IOS-CS results of Reid et al ., rate coefficients for a Maxwellian velocity distribution are computed and compared in Fig. 5 with total de-excitation measurements [29] , [30] , [31] reported by Reid et al . 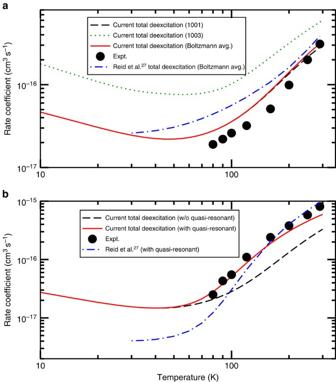Figure 5: Rate coefficients for the vibrational de-excitation of CO(v1=1) due to H2. Current 6D/CC (solid, dashed and dotted lines) and Reidet al.274D (dot-dashed line) calculations are compared with the total CO(v1=1) rovibrational quenching experiment (symbols)29,30,31. (a) Ortho-H2rate coefficients for initial state-resolved,, summed overand(dashed and dotted lines) and for a Boltzmann average of initial H2(j2=1,3) (solid and dot-dashed lines). (b) Para-H2rate coefficients for a Boltzmann average of initial H2(j2=0,2) with and without the quasi-resonant process (2). Note that the experimental uncertainties are smaller than the symbol sizes. [27] The comparison is not straight forward because (i) the measurements correspond to an initial thermal population of H 2 rotational states, (ii) the initial rotational population of CO( v 1 =1, j 1 ) was unknown, (iii) the experimental rate coefficients for ortho-H 2 are estimated from para- and normal-H 2 measurements and (iv) the contribution from a quasi-resonant channel, Figure 5: Rate coefficients for the vibrational de-excitation of CO( v 1 =1) due to H 2 . Current 6D/CC (solid, dashed and dotted lines) and Reid et al . [27] 4D (dot-dashed line) calculations are compared with the total CO( v 1 =1) rovibrational quenching experiment (symbols) [29] , [30] , [31] . ( a ) Ortho-H 2 rate coefficients for initial state-resolved, , summed over and (dashed and dotted lines) and for a Boltzmann average of initial H 2 ( j 2 =1,3) (solid and dot-dashed lines). ( b ) Para-H 2 rate coefficients for a Boltzmann average of initial H 2 ( j 2 =0,2) with and without the quasi-resonant process (2). Note that the experimental uncertainties are smaller than the symbol sizes. Full size image dominates the para-H 2 case for T ≳ 50 K. Figure 5a displays the CO( v 1 =1) rovibrational de-excitation rate coefficients from the current 6D/CC calculations for collisions of ortho-H 2 for j 2 =1 and 3, separately. These rate coefficients are summed over all and . Assuming a Boltzmann average at the kinetic temperature T of the H 2 rotational levels j 2 =1 and 3, presumed to be representative of the experimental conditions, rate coefficients are computed and found to be in good agreement with the measurements above 200 K. From Fig. 5a , the contribution from j 2 =3 is seen to be only important above 150 K. The remaining difference with experiment at low temperatures may be due to the fact mentioned above that the ortho-H 2 rate coefficients are not directly measured, but deduced from normal-H 2 and para-H 2 experiments. In particular, Reid et al . [27] assume that the ortho/para ratio in the normal-H 2 measurements is 3:1, that is, statistical, and independent of temperature. Further, as stated above, the experimental CO rotational population distribution in v 1 =1 is unknown. Nevertheless, the current 6D/CC computations are a significant advance over the 4D results of Reid et al . [27] , which also correspond to a Boltzmann average of rate coefficients for j 2 =1 and 3. As indicated above, the situation for para-H 2 collisions is more complicated due to the quasi-resonant contribution (2), a mechanism not important for ortho-H 2 . Boltzmann-averaged rate coefficients are presented in Fig. 5b including j 2 =0 and 2 summed over , with and without the quasi-resonant contribution, . While the current 6D/CC results and the 4D calculations of Reid et al . [27] are in agreement that the quasi-resonant contribution becomes important for T ≳ 50 K, the relative magnitude compared with the non-resonant transitions from the 6D/CC calculation is somewhat less than obtained previously with the 4D potential. This is partly related to the fact that the 6D/CC rate coefficients for j 2 =0 are significantly larger than those of Reid et al . [27] (see also the corresponding cross-sections in Fig. 4 and in the Supplementary Fig. 9 ). Compared with the experiment, we obtain excellent agreement for T ≲ 150 K, but are somewhat smaller at higher temperatures. This small discrepancy may be related to the unknown CO( v 1 =1, j 1 ) rotational population in the measurement. Nevertheless, it is only the 6D/CC computations, that is, dynamics in full dimensionality with full angular momentum coupling, that can reproduce the measurements for both ortho- and para-H 2 . Further, the computations for the quasi-resonant process (2) were the most challenging reported here due to the requirement of a very large basis set (see Supplementary Table 2 ), which resulted in long computation times, a large number of channels and usage of significant disk space (~0.5 TB per partial wave). In total, the cross-sections given here consumed >40,000 CPU hours. The current investigation of the CO–H 2 inelastic collision system has been performed with the intent of minimal approximation through the computation of a high-level PES, robust surface fitting and full-dimensional inelastic dynamics with full angular momentum coupling. That is, within this paradigm for studying inelastic dynamics, we have advanced the state-of-the-art for diatom–diatom collisions through this unprecedented series of computations. The approach has been benchmarked against experiment for pure rotational and rovibrational transitions giving the most accurate results to date within the experimental uncertainties and unknowns. The accuracy and long-range behaviour of the 6D PES is found to be comparable to previous, lower-dimensional surfaces. The agreement of the current computation for the CO( v 1 =1) rovibrational quenching with measurement resolves a long-standing (more than two-decades) discrepancy and justifies the requirement of a full-dimensional approach. This methodology can now, though with significant computational cost, be applied to a large range of initial rotational levels for v 1 =1 and for higher vibrational excitation to compute detailed state-to-state cross-sections unobtainable via experiment. This advance in computational inelastic scattering is particularly timely as ground-based (for example, the Very Large Telescope (VLT)) observations have focused on CO rovibrational emission/absorption in a variety of astrophysical objects, while related observations are in the planning stages for future space-based telescopes (for example, NASA’s James Webb Space Telescope). In particular, we are in an exciting era of investigation into the properties of PPDs around young stellar objects [47] . PPDs provide the material for newly forming stars and fledgling planets. The CO fundamental band (|Δ v 1 |=1) is a tracer of warm gas in the inner regions of PPDs and, with appropriate modelling, gives insight into disk-gas kinematics and disk evolution in that zone where planets are expected to be forming. A recent survey of 69 PPDs with the VLT [19] detected CO vibrational bands in 77% of the sources including v 1 =1→ 0, v 1 =2→1, v 1 =3→2, and even v 1 =4→3 in a few cases. Remarkably, rotational excitation as high as j 1 =32 was observed. However, the modelling of PPDs, and other astrophysical sources with CO vibrational excitation, is hindered by the lack of rate coefficients due to H 2 collisions. We are now in an excellent position to provide full-dimensional, state-to-state CO–H 2 collisional data, which will not only have a profound impact on models characterizing these intriguing environments that give birth to planets, but also aid in critiquing current theories used to describe their evolution. Potential energy computations The potential energy computations were performed using the explicitly correlated coupled cluster (CCSD(T)-F12b) method [48] , [49] , as implemented in MOLPRO2010.1 (ref. 50 ). The cc-pcvqz-f12 orbital basis sets [51] that have been specifically optimized for use with explicitly correlated F12 methods and for core-valence correlation effects have been adopted. Density fitting approximations [49] were used in all explicitly correlated calculations with the AUG-CC-PVQZ/JKFIT and AUG-CC-PWCVQZ-MP auxiliary basis sets [52] , [53] . The diagonal, fixed amplitude 3C(FIX) ansatz was used, which is orbital invariant, size consistent, and free of geminal basis set superposition error (BSSE) [54] , [55] . The default CCSD-F12 correlation factor was employed in all calculations, and all coupled cluster calculations assume a frozen core (C:1 s and O:1 s). The counter-poise (CP) correction [56] was employed to reduce BSSE. Although the explicitly correlated calculations recover a large fraction of the correlation energy, the CP correction is still necessary, mainly to reduce the BSSE of the Hartree–Fock contribution. Benchmark calculations at the CCSD(T)-F12b/cc-pcvqz-f12 level were carried out on selected molecular configurations and results were compared with those from the conventional CCSD(T) method using aug-cc-pV5Z and aug-cc-pV6Z basis sets. Results showed that the CP-corrected interaction energy agrees closely with those derived from CCSD(T)/aug-cc-pV6Z. To construct the PES, the computations were performed on a six-dimensional (6D) grid using Jacobi coordinates as shown in Supplementary Fig. 1 . R is the distance between the centre of mass of CO and H 2 . r 1 and r 2 are the bond lengths of CO and H 2 , respectively. θ 1 is the angle between r 1 and R , θ 2 the angle between r 2 and R , and φ the out-of-plane dihedral or twist angle. In the potential energy computations, the bond lengths are taken over the ranges 1.7359 ≤ r 1 ≤ 2.5359 a 0 and 1.01 ≤ r 2 ≤ 1.81 a 0 , both with a step-size of 0.1 a 0 . For R , the grid extends from 4.0 to 18.0 a 0 with step-size of 0.5 a 0 for R < 11.0 a 0 and 1.0 a 0 for R > 11.0 a 0 . All angular coordinates were computed with a step-size of 15° with 0 ≤ θ 1 ≤ 360° and 0 ≤ θ 2 , φ ≤ 180°. Additional points were added in the region of the van der Waals minimum. The PES fit The CO–H 2 interaction PES has been fitted in 6D using an invariant polynomial method [37] , [38] . The PES was expanded in the form, where y i = e - 0.5 d i is a Morse-type variable. The internuclear distances d i between two atoms are defined as d 1 = d HH' , d 2 = d OH' , d 3 = d CH' , d 4 = d CH , d 5 = d OH and d 6 = d CO . The total power of the polynomial, N = n 1 + n 2 + n 3 + n 4 + n 5 + n 6 , was restricted to a maximum of 6. Expansion coefficients c n 1 . . . n 6 were obtained using weighted least-squares fitting for potential energies up to 10,000 cm −1 . The RMS error in the fit of the PES is 14.22 cm −1 , which included 398,218 different geometries. This RMS error can be compared with that of 277 cm −1 for the 6D reactive surface of Zhang et al . [36] which, however, extended to more than 30,000 cm −1 . From the computed energy points, the global minimum of the total potential corresponds to the collinear arrangement H-H-C-O ( θ 1 =0, θ 2 =0, φ =0) with a depth of −85.937 cm −1 at R =8.0 a 0 with r 1 and r 2 at their, respectively, equilibrium positions. This compares with the global minimum of the interaction potential obtained by Jankowski et al . [35] from their fitted V12 PES averaged over r 1 and r 2 : R =7.911 a 0 and −93.651 cm −1 . Note that this comparison is only suggestive, as the global minimum in the total and interaction potentials coincide only when bond lengths ( r 1 and r 2 ) are fixed at their equilibrium values as illustrated in Fig. 1 and that is not the case for V12. Scattering theory and computational details The quantum scattering theory for a collision of an S -state atom with a rigid-rotor was developed [2] , [57] , [58] , [59] , based on the close-coupling (CC) formulation of Arthurs and Dalgarno [1] . Details about its extension to diatom–diatom collisions with full-vibrational motion can be found in refs 12 , 13 . In this approach, the interaction potential V ( R , r 1 , r 2 , θ 1 , θ 2 , φ ) is expanded as, with the bi-spherical harmonic function expressed as, where 0 ≤ λ 1 ≤ 10, 0 ≤ λ 2 ≤ 6 was used in the scattering calculations. Owing to the symmetry of H 2 , only even values of λ 2 contribute. For convenience, the combined molecular state (CMS) notation is applied to describe a combination of rovibrational states for the two diatoms. A CMS represents a unique quantum state of the diatom–diatom system before or after a collision. The CMS will be denoted as ( v 1 j 1 v 2 j 2 ). v and j are the vibrational and rotational quantum numbers. The rovibrational state-to-state cross-section as a function of collision energy E is given by, where ( v 1 j 1 v 2 j 2 ) and ( ) are, respectively, the initial and final CMSs of CO–H 2 , the wave vector k 2 =2 μE / ℏ 2 and S is the scattering matrix. l is the orbital angular momentum and J the total collision system angular momentum, where J = l + j 12 and j 12 = j 1 + j 2 . Thorough convergence testing was performed in the scattering calculations by varying all relevant parameters. The CC equations were propagated for each value of R from 4 to 18.0 a 0 using the log-derivative matrix propagation method of Johnson [60] and Manolopoulos [61] , which was found to converge for a radial step-size of Δ R =0.05 a 0 . The convergence tests of the v 1 = 1 → 0 vibrational quenching cross-section of CO with respect to the number of v 1 =1 rotational channels found that at least 13–15 channels have to be included in the v 1 =1 basis set, especially for low-energy scattering. On the basis of convergence tests with respect to the adopted maximum R for the long-range part of the PES, we found that the cross-sections are converged down to the lowest collision energy of 0.1 cm −1 . This value also guarantees that the rate coefficients are converged for temperatures >1 K. The number of discrete variable representation points N r 1 and N r 2 ; the number of points in θ 1 and θ 2 for Gauss-Legendre quadrature, N θ 1 and N θ 2 ; and the number of points in φ for Gauss-Hermite quadrature, N φ , which were applied to project out the potential expansion coefficients, were all tested for convergence with the final adopted values given in Supplementary Table 2 . The basis sets and the maximum number of coupled channels are also presented in Supplementary Table 2 . The resulting integral cross-sections were thermally averaged over a Maxwellian kinetic energy distribution to yield state-to-state rate coefficients as function of temperature T , where m is the reduced mass of the CO–H 2 complex, β =( k B T ) −1 and k B is Boltzmann’s constant. How to cite this article: Yang, B.H. et al . Quantum dynamics of CO-H 2 in full dimensionality. Nat. Commun. 6:6629 doi: 10.1038/ncomms7629 (2015).